Engineering the architectural diversity of heterogeneous metallic nanocrystals Similar to molecular engineering where structural diversity is used to create more property variations for application explorations, the architectural engineering of heterogeneous metallic nanocrystals (HMNCs) can likewise increase the versatility of metallic nanocrystals (NCs). Here we present a synthesis strategy capable of engineering the architectural diversity of HMNCs through rational and independent programming of every architecture-determining element, that is, the shape and size of the component NCs and their spatial arrangement. The strategy is based on the galvanic replacement reaction of a self-sustaining layer formed by underpotential deposition on a polyhedral NC. The selective deposition of satellite NCs on specific site of the central NC is realized by creating a geometry-dependent heterogeneous electron distribution. This site-selective deposition approach is applicable to central NCs in various polyhedral shapes and sizes. The satellite NCs can further develop their own shape and size through crystal growth kinetics control. The development of a diversity of materials with the desired functionalities and performance from a limited number of elements provided by nature has always been the challenge for chemists and material scientists. To this end, the organic chemists have done very well—for they have crafted numerous organic molecules from basic elements such as carbon, hydrogen and oxygen by changing the number and the type of atoms and their spatial relationship. Taking a lesson from such an approach, we developed a synthesis strategy capable of engineering the architecture of heterogeneous metallic nanocrystals (HMNCs) through rational and independent programming of every architecture-determining element of a HMNC, that is, the shape and size of the component nanocrystals (NCs) and their spatial arrangement ( Fig. 1 ). Architectural engineering of HMNCs can generate metallic nanostructures with unprecedented diversity and structural complexity mimicking those of organic molecules (see Supplementary Figs S1 and S2 and Supplementary Note 1 ). Integrating different metallic NCs into a HMNC can introduce new and enhanced properties, or multi-functionality not found in the parent metal NCs [1] , [2] , [3] , [4] , [5] , [6] , [7] . The properties of a HMNC are clearly architecture dependent [7] , [8] , [9] , [10] , [11] , [12] , [13] , [14] , [15] , [16] , [17] . Therefore, architectural engineering of HMNCs can significantly increase the possibilities to create new and more varied properties for application explorations. 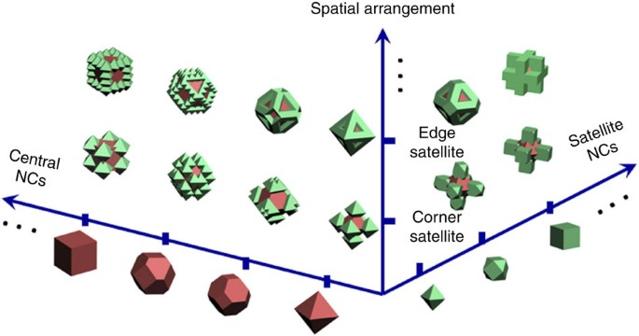Figure 1: Schematic illustration of the architectural diversity of binary HMNCs. The three axes represent the architecture-determining elements of a HMNC, namely, the geometries of central and satellite NCs and their relative spatial arrangement. The HMNC examples shown here are formed by the selective deposition of satellite NCs on the corners or edges of the central NC. The morphology of both the central and satellite NCs can be varied to have the NC-exposed surface bound by {111}, {100} or a combination of both. Figure 1: Schematic illustration of the architectural diversity of binary HMNCs. The three axes represent the architecture-determining elements of a HMNC, namely, the geometries of central and satellite NCs and their relative spatial arrangement. The HMNC examples shown here are formed by the selective deposition of satellite NCs on the corners or edges of the central NC. The morphology of both the central and satellite NCs can be varied to have the NC-exposed surface bound by {111}, {100} or a combination of both. Full size image Our strategy leverages on several concepts central to the rational and independent programming of the shape and size of central and satellite NCs, and their spatial relationship in a HMNC. The most unique features of our strategy are the generation of a geometry-dependent heterogeneous electron distribution by a smart chemical reaction system (vide infra) to induce the site-selective deposition of satellite NCs on a polyhedral central NC; and tuning the electron distribution by the kinetics of electron generation to alter the deposition sites on the central NC. This selective deposition of satellite NCs on the desired sites of a polyhedral central NC is universal and applies to polyhedral central NCs in various shapes and sizes; and preserves the geometric invariance of the latter throughout the course of satellite NC deposition. In addition, the crystal growth kinetics may be varied over a broader range of values to provide shape and size customizability of the satellite NCs without affecting the deposition sites. Principles The site-selective deposition is accomplished by a facile smart chemical reaction system based on the galvanic replacement reaction of a metal layer formed sustainably by underpotential deposition (UPD) on a central NC. We will use binary Au/AgPd HMNCs consisting of an Au central NC and bimetallic AgPd satellite NCs to demonstrate the synthesis strategy ( Fig. 2 ). In this approach, UPD is used to reverse the order of the reduction potentials of the two metal precursors (Ag and Pd precursors). The precursor of the more reactive metal (Ag in this case) is quickly reduced to form a Ag UPD layer on the central NC [18] , [19] , [20] , [21] , [22] , [23] , which would otherwise be the less favourable metal for reduction without UPD ( Fig. 2i-ii ). This in-situ formed Ag UPD layer then undergoes galvanic replacement reaction with the precursor of the less reactive metal (Pd precursor in this case) because of the difference in their reduction potentials [24] ( Fig. 2iii ). The electrons released from the galvanic replacement reaction then accumulate preferentially on certain NC sites [25] , [26] , [27] , [28] , [29] . In this way, a spatially heterogeneous electron distribution is created, which can be used to direct the deposition of satellite NCs on electron-rich sites. It should be mentioned that the Ag UPD layer is self-sustaining. Once the Ag atoms in the Ag UPD layer are oxidized and dissolved away, the exposure of the underlying central NC will again induce the UPD of Ag to replenish the Ag UPD layer lost to galvanic oxidation ( Fig. 2iv ). The persistence of the Ag layer due to a fast UPD and its simultaneous galvanic oxidation provide a steady and continuous supply of electrons to specific regions on the central NC surface ( Fig. 2iii-iv ). These are the basis for maintaining a distributed presence of satellite NCs on the central NC ( Fig. 2v ). 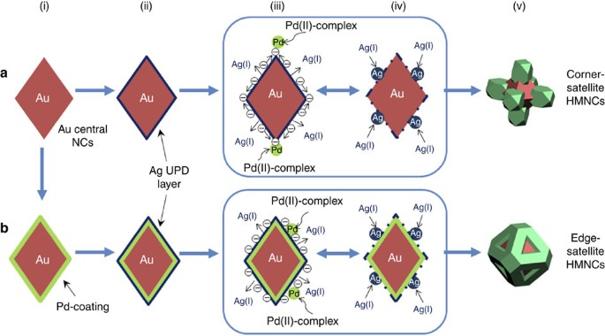Figure 2: Schematic illustrations of corner- and edge-selective depositions by the strategy of this study. The corner- and edge-selective depositions are shown in rowsaandb, respectively. (i) Au central NCs in a well-defined morphology were prepared. (ii) The Ag precursor was reduced first due to UPD and quickly formed a Ag monolayer on the central NCs. (iii) Thisin situformed Ag layer then underwent galvanic replacement reaction with the Pd precursor due to the difference in their reduction potentials. The electrons released by the galvanic oxidation of the Ag layer then travelled to and accumulated at the corners (a) or the edges (b) of the Au central NCs because of the high curvatures there. The Pd precursor would be reduced and deposited preferentially on these electron-rich regions. (iv) The Ag layer was self-sustaining due to the swiftness of UPD, that is, once the Ag atoms in the Ag layer were oxidized and dissolved, UPD of Ag would immediately occur to replenish the Ag atoms lost to oxidation. The newly formed Ag UPD layer would then be oxidized and regenerated. The cycle went on (the boxed regions in iii and iv). (v) This cyclic process ensured a continuous supply of electrons to the corners of the central NC to sustain the reduction there. For the preparation of edge-satellite HMNCs, the surface of the Au central NCs was modified by Pd-coating (b(i)), and a Ag layer was formed on the Pd-coated Au NCs (b(ii)). Figure 2: Schematic illustrations of corner- and edge-selective depositions by the strategy of this study. The corner- and edge-selective depositions are shown in rows a and b , respectively. (i) Au central NCs in a well-defined morphology were prepared. (ii) The Ag precursor was reduced first due to UPD and quickly formed a Ag monolayer on the central NCs. (iii) This in situ formed Ag layer then underwent galvanic replacement reaction with the Pd precursor due to the difference in their reduction potentials. The electrons released by the galvanic oxidation of the Ag layer then travelled to and accumulated at the corners ( a ) or the edges ( b ) of the Au central NCs because of the high curvatures there. The Pd precursor would be reduced and deposited preferentially on these electron-rich regions. (iv) The Ag layer was self-sustaining due to the swiftness of UPD, that is, once the Ag atoms in the Ag layer were oxidized and dissolved, UPD of Ag would immediately occur to replenish the Ag atoms lost to oxidation. The newly formed Ag UPD layer would then be oxidized and regenerated. The cycle went on (the boxed regions in iii and iv). (v) This cyclic process ensured a continuous supply of electrons to the corners of the central NC to sustain the reduction there. For the preparation of edge-satellite HMNCs, the surface of the Au central NCs was modified by Pd-coating ( b (i)), and a Ag layer was formed on the Pd-coated Au NCs ( b (ii)). Full size image Controlling the spatial relationship of component NCs This site-selective deposition approach is based on the manoeuvrability of electron distribution on a polyhedral NC surface. We were able to direct the electron flow to the corners or the edges of the polyhedral central NC to form corner-/edge-satellite HMNCs. Corners and edges are the defining features of any polyhedron. The ability to position satellite NCs exclusively on the corners or edges can be used to create a large library of well-defined HMNC architectures. 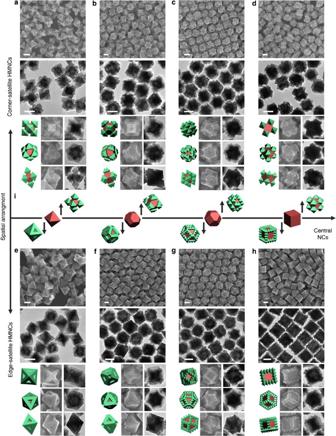Figure 3: Tuning of the spatial arrangement of the component NCs and the shape of the central NCs in Au/AgPd HMNCs. (a–d) Corner-satellite HMNCs and (e–h) edge-satellite HMNCs. The central NCs are (a,e) octahedrons, truncated octahedrons with (b,f) small and (c,g) large truncation degrees, and (d,h) cubes. The satellite NCs are all bound by {111} facets. The images in each panel are arranged from top to bottom to include the scanning electron microscopy (SEM) images, the transmission electron microscopy (TEM) images and the geometric models (and associated SEM and TEM images) of an individual HMNC viewed from the <100>, <111> and <110> directions. (i) Schematic illustration of the HMNCs formed by tuning the polyhedral shape of the central NCs (horizontal axis) and the spatial arrangement (vertical axis, upward for corner-satellite HMNCs and downward for edge-satellite HMNCs). Scale bars, 50 nm. Figure 3 and Supplementary Figs S3–S9 show the selective deposition of satellite NCs on the corners or the edges of some example polyhedral central NCs (see Supplementary Notes 2 and 3 for the detailed structural analysis). It is well known that the free charges on the surface of a conductor would move preferentially to high curvature sites. Corners and edges are the high curvature sites of a polyhedron, where electrons would accumulate. The distribution of electrons can be altered by controlling the kinetics of electron generation. A slow electron generation rate allows the electrons to accumulate only in regions of the highest curvature, that is, corners of the polyhedral central NC. On the other hand, a faster electron generation rate can disperse the electrons over a wider area, although regions of high curvature are still preferred. In this case, the electrons could congregate along the edges. As the electrons are generated by the galvanic oxidation of the Ag layer, the rate of electron generation can be moderated by making adjustments to the reactivity (oxidizability) of the Ag layer. This is most easily done by modifying the surface properties of the central NC on which the Ag layer is formed. The central NC, as the substrate of the Ag layer, can cause lattice strain in the Ag layer to affect the Ag reactivity [30] . The surface of the central NCs can be modified by changing the addition sequence of the two metal precursors. A Ag layer is then formed either directly on the Au central NCs [18] , [19] , [20] , [21] or on Pd-coated Au central NCs ( Supplementary Note 4 and Supplementary Fig. S10 ). Pd-coating of the Au central NCs can result in more facile electron generation kinetics owing to the greater lattice mismatch between Ag and Pd (5.14 versus 0.02% between Ag and Au). The greater strain in the Ag layer formed on the Pd surface would increase the Ag reactivity, making Ag on Pd more oxidizable than Ag on Au. A slow Ag oxidation on the surface of the Au central NCs confines the deposition to the corners exclusively, whereas the increased rate of electron generation from Ag layer oxidation on Pd-coated Au central NCs allows the deposition of satellite NCs to occur on the edges ( Supplementary Note 5 and Supplementary Figs S11 and S12 ). Figure 3: Tuning of the spatial arrangement of the component NCs and the shape of the central NCs in Au/AgPd HMNCs. ( a – d ) Corner-satellite HMNCs and ( e – h ) edge-satellite HMNCs. The central NCs are ( a , e ) octahedrons, truncated octahedrons with ( b , f ) small and ( c , g ) large truncation degrees, and ( d , h ) cubes. The satellite NCs are all bound by {111} facets. The images in each panel are arranged from top to bottom to include the scanning electron microscopy (SEM) images, the transmission electron microscopy (TEM) images and the geometric models (and associated SEM and TEM images) of an individual HMNC viewed from the <100>, <111> and <110> directions. ( i ) Schematic illustration of the HMNCs formed by tuning the polyhedral shape of the central NCs (horizontal axis) and the spatial arrangement (vertical axis, upward for corner-satellite HMNCs and downward for edge-satellite HMNCs). Scale bars, 50 nm. Full size image Shape tuning of central NCs Our corner-/edge-selective deposition strategy is universally applicable to central NCs in various polyhedral shapes. Octahedrons, truncated octahedrons with different truncation degrees and cubes ( Supplementary Fig. S13 ) were used as the central NCs to form HMNCs in this study. These polyhedral central NCs have corners and edges in different sharpness or come in quasi-spherical shapes with relatively blunt corners and edges. They also possess different exposed crystallographic facets. Regardless of the polyhedral geometry of the central NCs, the satellite NCs were deposited only on the corners or along the edges as shown in Fig. 3 and Supplementary Figs S3–S9 . Such display of site selectivity regardless of the shape of the central NC is the result of curvature-directed electron distribution and demonstration of the uniqueness and general utility of this synthesis strategy. The corners and edges are of higher curvatures than the facets of any polyhedron and are therefore regions of electron accumulation. The central NCs with well-developed polyhedral shapes were prepared in a separate step and are inert to the galvanic replacement reaction. Their geometry could be independently varied and preserved throughout the process. The central NC therefore operates as a template to transfer the desired geometrical features to the UPD Ag layer to start the site-specific deposition. Shape tuning of satellite NCs The satellite NCs in both corner- and edge-satellite HMNCs can develop their own morphology without changes in the deposition sites. This is distinctly shown by examples of HMNCs with satellite NCs bound by low-index {111} ( Fig. 3 ), {100} facets or a combination of both ( Fig. 4 and Supplementary Figs S14–S18 ; see Supplementary Notes 6 and 7 for the detailed structural and compositional analyses). A NC shape can be tuned by the careful control of the crystal growth kinetics, that is, the relative growth rates in different crystallographic directions during crystal growth [25] , [31] , [32] . The reaction conditions in the synthesis can be used to alter the crystal growth kinetics of the satellite NCs without changing their deposition sites so long as there is sustained Ag layer formation and oxidization to supply the electrons for the deposition of satellite NCs on specific sites. The shape of the satellite NCs can be varied by the [Ag + ]/[Pd 2+ ] concentration ratio and the concentration of HCl (which is used as an additive). These preparation variables are able to modify the preferred growth directions of the metal atoms [33] or the reduction rates of their precursors [10] , [34] to yield different shapes of satellite NCs. 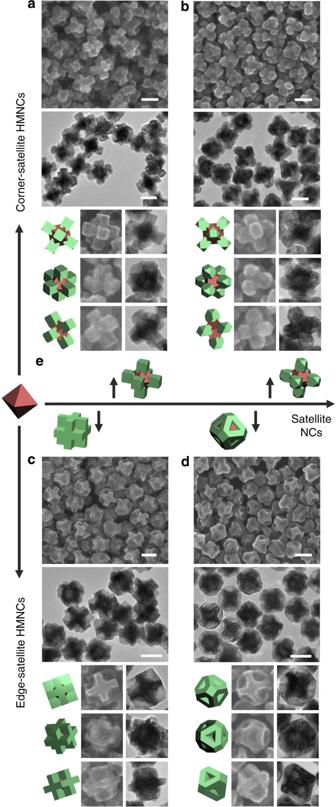Figure 4: Tuning the shape of satellite NCs in Au/AgPd HMNCs. The satellite NCs are bound by (a,c) {100} facets and (b,d) {100} and {111} facets. (a,b) Corner-satellite HMNCs and (c,d) edge-satellite HMNCs. The central NCs are octahedrons. The images in each panel are arranged from top row to bottom to include the SEM images, the TEM images and the geometric models (and associated SEM and TEM images) of an individual HMNC viewed from the <100>, <111> and <110> directions. (e) Schematic illustration of the corner-satellite (upward vertical axis) and edge-satellite (downward vertical axis) HMNCs formed by tuning the polyhedral shape of the satellite NCs (horizontal axis). Scale bars, 50 nm. Figure 4: Tuning the shape of satellite NCs in Au/AgPd HMNCs. The satellite NCs are bound by ( a , c ) {100} facets and ( b , d ) {100} and {111} facets. ( a , b ) Corner-satellite HMNCs and ( c , d ) edge-satellite HMNCs. The central NCs are octahedrons. The images in each panel are arranged from top row to bottom to include the SEM images, the TEM images and the geometric models (and associated SEM and TEM images) of an individual HMNC viewed from the <100>, <111> and <110> directions. ( e ) Schematic illustration of the corner-satellite (upward vertical axis) and edge-satellite (downward vertical axis) HMNCs formed by tuning the polyhedral shape of the satellite NCs (horizontal axis). Scale bars, 50 nm. Full size image Size tuning of HMNCs The size of the central and satellite NCs can also be independently varied while keeping their shape and deposition sites unchanged. We will use corner-satellite HMNCs with octahedral central and satellite NCs to demonstrate this size tunability. The satellite NCs were able to retain their octahedral shape and corner deposition, whereas their size was varied, as shown in Fig. 5a–c . Such size tuning is independent of the size of the central NC. Hence, the size of HMNCs can be varied without affecting their overall architecture if the size ratio of satellite to central NCs is kept the same, as shown in Fig. 5d–f . For size tuning, the central NCs were prepared in several discrete sizes ( Supplementary Fig. S19 ); the size of the satellite NCs was controlled by regulating the concentration ratios of the metal precursors to the central NCs. The deposition site and the shape of the satellite NCs were unchanged as long as the reaction conditions could sustain the deposition and oxidation of the Ag layer; and promote the crystal growth kinetics favourable for the development of the desired satellite NC shape. 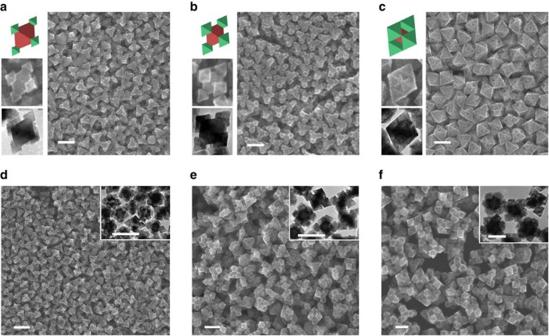Figure 5: Tuning the size of Au/AgPd HMNCs. (a–c) SEM images of Au/AgPd HMNCs with satellite NCs in various sizes. Insets show the geometrical models, SEM and TEM images of corresponding individual HMNC viewed along the <110> direction. The satellite NCs have edge length of (a) 25, (b) 30 and (c) 45 nm. (d–f) SEM images of Au/AgPd HMNCs in various sizes with inset showing corresponding TEM images. The distance between two furthest tips of the HMNCs is (d) 75, (e) 110 and (f) 150 nm. Scale bars, 100 nm. Figure 5: Tuning the size of Au/AgPd HMNCs. ( a – c ) SEM images of Au/AgPd HMNCs with satellite NCs in various sizes. Insets show the geometrical models, SEM and TEM images of corresponding individual HMNC viewed along the <110> direction. The satellite NCs have edge length of ( a ) 25, ( b ) 30 and ( c ) 45 nm. ( d – f ) SEM images of Au/AgPd HMNCs in various sizes with inset showing corresponding TEM images. The distance between two furthest tips of the HMNCs is ( d ) 75, ( e ) 110 and ( f ) 150 nm. Scale bars, 100 nm. Full size image General utility and extension of strategy The general utility of our strategy to site- and shape-selective synthesis of HMNCs was also tested on other metallic systems. We will use HMNCs consisting of Au central NCs and AgPt satellite NCs as an example. UPD of Ag layer on the Au octahedral NCs occurred similarly as in the preparation of Au/AgPd HMNCs. Different from the latter, the Ag layer underwent galvanic replacement reaction with the Pt precursor in this case. Both the deposition site (corner-satellite) and the shape (quasi-octahedral) of the AgPt satellite NCs could be controlled very well, as shown in Fig. 6a and Supplementary Fig. S20 . The synthesis approach is therefore versatile enough to produce many HMNCs with programmable architectures. 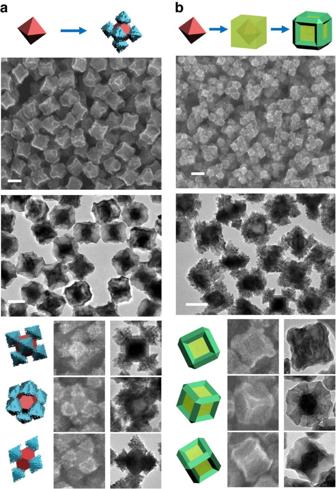Figure 6: General utility and extension of strategy. (a) Architectures of corner-satellite Au/AgPt HMNCs with AgPt bimetallic satellite NCs. (b) Architectures of ternary Au/Pd/AgPd HMNCs with a central Au NC, cubic Pd shell and satellite AgPd NCs on the edges of the Pd shell. Each panel contains, from top to bottom, the geometric models of the central NCs and corresponding HMNCs, SEM images, TEM images and the geometric models and associated SEM and TEM images of an individual HMNC viewed from the <100>, <111> and <110> directions. Scale bars, 50 nm. Figure 6: General utility and extension of strategy. ( a ) Architectures of corner-satellite Au/AgPt HMNCs with AgPt bimetallic satellite NCs. ( b ) Architectures of ternary Au/Pd/AgPd HMNCs with a central Au NC, cubic Pd shell and satellite AgPd NCs on the edges of the Pd shell. Each panel contains, from top to bottom, the geometric models of the central NCs and corresponding HMNCs, SEM images, TEM images and the geometric models and associated SEM and TEM images of an individual HMNC viewed from the <100>, <111> and <110> directions. Scale bars, 50 nm. Full size image Multi-component HMNCs, that is, HMNCs with more than two types of component NCs can also be fabricated. Figure 6b and Supplementary Fig. S21 are one example of ternary Au/Pd/AgPd HMNCs with Au octahedral central NCs overlaid with a cubic Pd shell ( Supplementary Fig. S22 ); and satellite AgPd NCs on the edges of the Pd shell. These multi-component HMNCs possess an even higher degree of architectural diversity, as each component NC, with its own morphology and spatial arrangement, can be combined in multiple ways to greatly increase the number of HMNC variants. We have developed a versatile synthesis strategy where every architecture-determining element of a HMNC may be systematically and independently varied to increase the structural diversity of HMNCs. This strategy takes advantage of the galvanic replacement reaction of a self-sustaining UPD layer on a central NC to generate a geometry-dependent heterogeneous distribution of electrons, and couples this with the tuning of crystal growth kinetics to enable independent size, shape and spatial relationship control for the central and satellite NCs. A large library of HMNCs with very diverse architectures can then be created by the rational programming of every architectural determining element of the HMNC. Such capability is immensely valuable to the development of architecture-dependent scaling laws and increases the possibilities to create new and more varied properties for application explorations. Materials Hydrogen tetrachloroaurate (Ш) hydrate (HAuCl 4 .xH 2 O, Alfa Aesar, 49.87% Au), palladium (II) chloride (PdCl 2 , Sigma-Aldrich, 98%), silver nitrate (AgNO 3 , Merck, 99.8%), sodium borohydride (NaBH 4 , Fluka, 98%), cetyltrimethylammonium bromide (Sigma-Aldrich, ≥98%) and L -ascorbic acid (Merck, 99%) were used as received. Ultrapure Millipore water (18.2 MΩ) was used as the solvent throughout. All glassware was cleaned in Aqua Regia and rinsed with ethanol and ultrapure water. A concentration of 5 mM H 2 PdCl 4 solution was prepared by dissolving 22.25 mg of PdCl 2 in 25 ml of 10 mM HCl solution. Synthesis of polyhedral Au NCs Au NCs in various polyhedral shapes (octahedrons, truncated octahedrons with different degrees of truncation and cubes) were prepared first and used as the central NCs for the preparation of HMNCs. The details in the preparation of these polyhedral Au NCs are given in Supplementary Methods . Synthesis of corner-satellite Au/AgPd HMNCs For the synthesis of corner-satellite Au/AgPd HMNCs with satellite NCs bound by {111} facets, 36 μl of 5 mM AgNO 3 (60 μl for cubic Au central NCs) and 0.155 ml of 38.8 mM ascorbic acid were added to 3 ml polyhedral Au NC solution. After thorough mixing, 60 μl of 100 mM HCl and specific volumes of 5 mM H 2 PdCl 4 were added to the polyhedral Au NC solution. The volume of H 2 PdCl 4 solution used for octahedral, truncated octahedral and cubic Au NC solutions was 42, 21 and 60 μl, respectively. The solutions were well mixed and left on the shaker overnight. For the synthesis of corner-satellite Au/AgPd HMNCs with satellite NCs bound by {100} or a combination of both {111} and {100} facets, only the amounts of AgNO 3 and HCl solutions were modified. Other reagents and experimental conditions were the same as those in the synthesis of satellite NCs bound by {111} facets. Satellite NCs bound by {100} facets were prepared by adding 60 μl of 0.5 mM AgNO 3 to the growth solution. Satellite NCs bound by both {100} and {111} facets were prepared by adding 60 μl of 0.5 mM AgNO 3 and 150 μl of 100 mM HCl to the growth solution. For the size tailoring of corner-satellite NCs bound by {111} facets on central octahedral NCs, the amounts of H 2 PdCl 4 and AgNO 3 solutions were modified, whereas other experimental variables remained constant. For the preparation of small satellite NCs, 9 μl and 21 μl of 5 mM H 2 PdCl 4 were added to the octahedral Au NC solution. For satellite NCs with larger sizes, the growth solution containing 60 μl of 5 mM AgNO 3 ; and 30 μl of 5 mM H 2 PdCl 4 was added to the growth solution twice at 30 min apart to prevent the self-nucleation of Pd NCs. For the size tailoring of the entire HMNCs, octahedral NCs in different sizes were used as the central NCs, whereas all other experimental conditions were unchanged. Synthesis of edge-satellite Au/AgPd HMNCs For the synthesis of edge-satellite Au/AgPd HMNCs with satellite NCs bound by {111} facets, 0.155 ml of 38.8 mM ascorbic acid, 60 μl of 100 mM HCl and 42 μl of 5 mM H 2 PdCl 4 were added to 3 ml polyhedral Au NC solution with thorough mixing after each addition. After aging the growth solution for 10 min, 36 μl of 5 mM AgNO 3 (60 μl for cubic Au central NCs) was added and mixed by shaking. Finally, 18 μl of 5 mM H 2 PdCl 4 was introduced 30 min after the AgNO 3 solution addition. The solution was thoroughly mixed and left on the shaker overnight. The amount of AgNO 3 solution was adjusted to produce edge-satellite NCs with other types of exposed facets. In particular, edge-satellite NCs bound by {100} facets or a combination of both {100} and {111} facets were obtained with 60 μl or 120 μl of 0.5 mM AgNO 3 added to the growth solution, respectively. All other experimental conditions remained the same. Materials characterizations The compositions and structures of central NCs and HMNCs were analysed by transmission electron microscopy (TEM), high-resolution TEM and energy-dispersive X-ray spectroscopy on JEM-2010 and JEM-2100F (JEOL) microscopes operating at 200 kV accelerating voltage. Field emission scanning electron microscopy (FESEM; on a JEOL JSM-6700F equipped with scanning TEM function operating at 25 kV) was used to evaluate overall particle morphology and product uniformity. TEM and SEM samples were typically prepared by dispensing a drop of the washed product on a copper grid followed by drying in air at room temperature. How to cite this article: Yu Y. et al. Engineering the Architectural Diversity of Heterogeneous Metallic Nanocrystals. Nat. Commun. 4:1454 doi: 10.1038/ncomms2474 (2013).